Regional boreal biodiversity peaks at intermediate human disturbance The worldwide biodiversity crisis has intensified the need to better understand how biodiversity and human disturbance are related. The 'intermediate disturbance hypothesis' suggests that disturbance regimes generate predictable non-linear patterns in species richness. Evidence often contradicts intermediate disturbance hypothesis at small scales, and is generally lacking at large regional scales. Here, we present the largest extent study of human impacts on boreal plant biodiversity to date. Disturbance extent ranged from 0 to 100% disturbed in vascular plant communities, varying from intact forest to agricultural fields, forestry cut blocks and oil sands. We show for the first time that across a broad region species richness peaked in communities with intermediate anthropogenic disturbance, as predicted by intermediate disturbance hypothesis, even when accounting for many environmental covariates. Intermediate disturbance hypothesis was consistently supported across trees, shrubs, forbs and grasses, with temporary and perpetual disturbances. However, only native species fit this pattern; exotic species richness increased linearly with disturbance. The ongoing human-caused global biodiversity decline and continuing expansion of human land use have deepened the need to better understand the relationship of biodiversity to anthropogenic disturbance [1] . The 'intermediate disturbance hypothesis' (IDH), a foundational idea in community ecology, suggests that differences in disturbance among local communities can explain broad patterns in diversity throughout a region [2] , [3] . In communities with moderate disturbance levels, species richness should be higher than in those with low or high disturbance [2] , [3] . After nearly 40 years of research, most studies have found little or no empirical evidence to support the IDH [4] . Support has been even slimmer with anthropogenic than with natural disturbances [4] , [5] , and our ability to predict changes in community diversity patterns following human disturbance is still extremely limited [4] , [5] . Further, studies of the IDH have rarely differentiated native and exotic species, a puzzling oversight given concerns of exotic species invasions, particularly in disturbed environments [6] . One reason implicated for the scarcity of empirical support for IDH [4] , [5] is that most investigations of diversity–disturbance relationships have been conducted at insufficiently small spatial scales [7] , [8] . Species richness varies non-linearly with spatial scale [9] , [10] , [11] and processes thought to generate IDH vary with scale [12] , so support for the IDH may itself depend on the scale at which it is tested [4] , [7] , [8] . Testing the IDH might best be accomplished by matching the scales of investigation to the scales at which those processes generating the IDH operate. Our understanding of the IDH is poorest at regional extents [4] , [5] (that is, across multiple landscapes), where it has been mostly limited to the system to which IDH was first applied, tropical forest trees. Further, at regional extents—those at which land use planning and management are often conducted—the IDH has generally been tested only with natural not anthropogenic disturbances [4] , [5] . We tested the specific prediction of the IDH that a non-linear unimodal relationship exists between species richness and anthropogenic disturbance extent, with the greatest number of species present at intermediate disturbance. We conducted our test by examining local communities across the largest spatial extent to date: the 381,047-km 2 boreal ecoregion of Alberta, Canada, an area comparable to Germany. Within this region, vascular plant species richness was sampled with 1 ha surveys of 242 local communities ( Fig. 1 ). We used a direct measure of anthropogenic disturbance: area of land altered by human land use (hereafter 'extent') as assessed with aerial and satellite imagery of 150 m radius circular areas. The sample plots exhibited a complete gradient (0–100%) in human disturbance extent: disturbances varied vastly in intensity, area and type among communities ranging from intact wilderness of one of the world's largest national parks (Wood Buffalo N.P.) to human-dominated landscapes of towns, forestry, agriculture, linear features, conventional oil and gas, and oil sands extraction. We found that species richness of boreal vascular plants showed a unimodal relationship with human disturbance. Richness peaked at intermediate disturbance, with or without accounting for numerous environmental factors, supporting the IDH. Also consistent with the IDH, communities at low and high human disturbance were composed of different sets of species, whereas communities with intermediate disturbance overlapped with those of low and high disturbance. However, we also tested the consistency of the IDH among native and exotic species individually and show that although native species exhibited the predicted peaked relationship of richness to human disturbance, exotic species instead increased linearly. 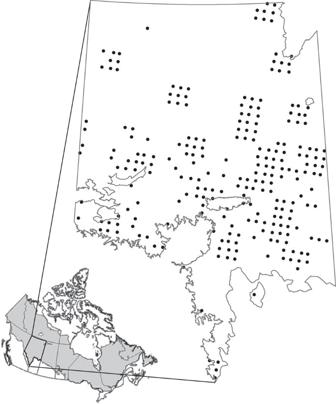Figure 1: Map of sampling locations. Presence of each vascular plant species was sampled at 242 sites within the boreal ecoregion of Alberta, Canada. The inset map shows Canada with the boreal region shaded. Figure 1: Map of sampling locations. Presence of each vascular plant species was sampled at 242 sites within the boreal ecoregion of Alberta, Canada. The inset map shows Canada with the boreal region shaded. Full size image Richness–disturbance relationship A simple unimodal model with peak at 47.7% disturbance best explained vascular plant species richness in relation to human disturbance extent: species richness peaked at intermediate disturbance ( Fig. 2 ), supporting the IDH. That simple quadratic curve ( r 2 =0.135, P <0.001, P of increase in r 2 over linear model <0.001) fit significantly better than other model shapes, whereas the linear regression model was not statistically significant ( r 2 =0.007, P =0.202; Supplementary Table S1 ). 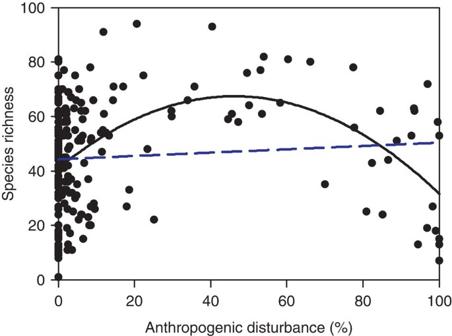Figure 2: Species richness to human disturbance relationship. Species richness per hectare of boreal vascular plants as a function of percent total anthropogenic disturbance extent. The black solid curve represents the adopted model, a quadratic curve (n=242,P<0.001), which supports the IDH. The blue dashed line represents another candidate model, a linear regression that was rejected. Figure 2: Species richness to human disturbance relationship. Species richness per hectare of boreal vascular plants as a function of percent total anthropogenic disturbance extent. The black solid curve represents the adopted model, a quadratic curve ( n =242, P <0.001), which supports the IDH. The blue dashed line represents another candidate model, a linear regression that was rejected. Full size image Species composition The IDH also predicts that composition of species should differ among communities depending on level of disturbance [2] , [3] . Mechanisms thought to drive the peaked disturbance–richness relationship, such as trade-offs in species traits associated with disturbance, suggest that communities with intermediate disturbance are more species rich because they are composed of species associated with both low and high disturbance levels [2] , [3] . Consistent with the IDH, we observed that communities with low (<33.3%) and high (>66.7%) disturbance were composed of significantly different sets of species ( P <0.001), with species composition overlapping least among communities of low and high disturbance ( A =0.028, Fig. 3 ). Also consistent with the IDH, species composition of communities with intermediate (33.4–66.6%) disturbance overlapped with composition of communities with low ( A =0.027) or high ( A =0.017) disturbance ( Fig. 3 ). The difference in composition between intermediate and low disturbance communities was statistically significant ( P <0.001), whereas the difference between intermediate and high disturbance communities was less clear: it was not significantly more different in species composition than would be expected by chance ( P =0.085), but the higher P -value may be due in part to fewer sites in that comparison. Although a high proportion of sites sampled exhibited low disturbance, 30.7% of species were found only at sites with <33.3% human disturbance. 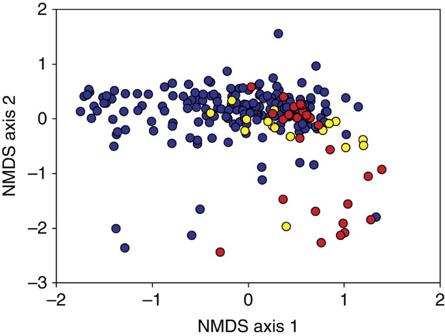Figure 3: Species composition compared by disturbance class. Non-metric multidimensional scaling (NMDS) ordination of species composition across sites. Each point represents a sample site and each site is classified by percent human disturbance (blue: <33.3%, yellow: 33.4–66.6%, red: >66.7%). Overlap of sites in different disturbance levels indicates similarity in species composition between those levels. The axes are unitless. Figure 3: Species composition compared by disturbance class. Non-metric multidimensional scaling (NMDS) ordination of species composition across sites. Each point represents a sample site and each site is classified by percent human disturbance (blue: <33.3%, yellow: 33.4–66.6%, red: >66.7%). Overlap of sites in different disturbance levels indicates similarity in species composition between those levels. The axes are unitless. Full size image Species origin and growth form One possible difference in species composition along the disturbance gradient is the proportion of native and exotic species. These groups are often managed differently: exotic species are traditionally considered of lesser conservation priority than native species and detrimental exotics ('invasive species') are often targets for control [13] . We therefore tested the IDH with native and exotic species separately. We found that although native species richness peaked at intermediate extent of human disturbance ( r 2 =0.104, P <0.001), exotic species richness increased linearly ( r 2 =0.371, P <0.001, P of increase in r 2 for quadratic model over linear=0.082, Fig. 4a ; Supplementary Table S2 ). As native and exotic species showed different shaped functions, we compared the changes in native and exotic richness at ranges in disturbance extent less than or greater than 'intermediate disturbance', where native richness peaked, to better understand relative changes in these species groups. At <47.7% disturbance extent, native species increased (linear regression slope=0.503) more steeply ( P =0.001, ANCOVA) with extent than exotic species (slope=0.119). However, at >47.7% disturbance extent, native species decreased (slope=−0.693, s.e.=0.172) significantly more steeply than exotic species increased (slope=0.022, s.e.=0.038) with disturbance, as indicated by the standard errors of the absolute values of the slopes that were less than the gap between those errors. Anthropogenic disturbance was a more accurate predictor of richness of exotic species than of natives; disturbance extent explained 3.6 times the variance in exotics than in natives ( Fig. 4a ). 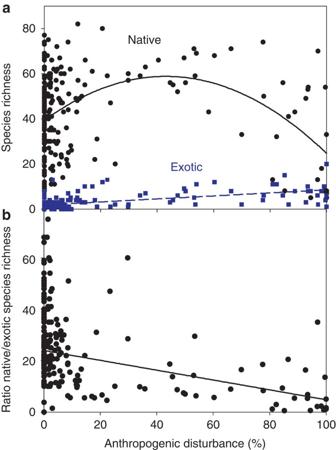Figure 4: Native and exotic species richness related to disturbance. Comparison of species richness per hectare of native and exotic boreal vascular plants in relation to percent anthropogenic disturbance extent. (a) Native (black circles) and exotic (blue squares) species richness as a function of disturbance extent. A quadratic model fit (solid black curve) native species richness with its peak at intermediate disturbance (n=237,P<0.001), whereas a linearly increasing model (dashed blue line) fit exotic species richness over human disturbance (n=237,P<0.001). (b) Ratio of native to exotic species richness as a function of disturbance extent decreased linearly. Figure 4: Native and exotic species richness related to disturbance. Comparison of species richness per hectare of native and exotic boreal vascular plants in relation to percent anthropogenic disturbance extent. ( a ) Native (black circles) and exotic (blue squares) species richness as a function of disturbance extent. A quadratic model fit (solid black curve) native species richness with its peak at intermediate disturbance ( n =237, P <0.001), whereas a linearly increasing model (dashed blue line) fit exotic species richness over human disturbance ( n =237, P <0.001). ( b ) Ratio of native to exotic species richness as a function of disturbance extent decreased linearly. Full size image The ratio of native to exotic species declined linearly with human-disturbed area (slope=−0.247, r 2 =0.203, P <0.001, Fig. 4b ). The IDH was conceived without apparent consideration of invasive species, and the non-conformance of exotics implies the hypothesis may only apply to regional metacommunities with a 'closed' species pool. The correlation of exotic species and human disturbance is consistent with previous studies [13] , and suggests that fundamentally different responses to disturbance exist among some groups. However, when we categorized species by 'growth form' [14] , another common ecological categorization and indicator of functional role, richness of each type of vascular plant species (including forbs, graminoids, shrubs and trees), peaked at intermediate disturbance extent ( Supplementary Table S3 ). The generality of the IDH among types of species requires greater scrutiny. Environmental covariates Total species richness varied considerably along the disturbance gradient, an expected result shared by other related observational studies [4] , [5] , [15] owing to effects of numerous other factors including climate, topography, stand age, soil and other environmental conditions. We accounted for many such factors by constructing multiple regression models that included 19 environmental variables ( Supplementary Table S4 ) including human disturbance, and again compared possible shapes of the relationship between richness and human disturbance. Consistent with the IDH, a quadratic curve with maximum species richness at intermediate disturbance fits best ( P <0.001, Supplementary Table S5 ). As expected, including the environmental variables in the model better explained species richness across sites ( r 2 =0.709) than did the simple quadratic model of human disturbance in response to richness ( r 2 =0.137, P =0.780; Supplementary Table S5 ). However, accounting for these variables did not qualitatively change the shape of the relationship between richness and disturbance. Anthropogenic disturbance types Anthropogenic disturbance varied greatly in intensity, frequency, permanence and spatial characteristics, so different types of disturbance might be expected to drive different disturbance–diversity relationships as a result. Agricultural disturbance is often so frequent and intensive (for example, annual cultivation) such that successional processes are minimal, and primary roads plus urban and industrial sites are virtually permanent landscape changes. We classified those disturbances as 'perpetual'. By contrast, vegetation on forestry cut blocks, pipelines and seismic lines usually exhibit dynamic and successional changes in species composition following initial disturbance, classified here as 'temporary'. To investigate the relationship of richness to proportion of temporary human footprint, we excluded perpetual human footprint. In areas not perpetually disturbed, richness again peaked at intermediate temporary disturbance extent. The simple quadratic model with peak at 55.3% temporary disturbance fit significantly better than other model shapes ( r 2 =0.1136, P <0.001, P of increase in r 2 over linear model <0.001; Supplementary Table S6 ); the linear model had a likelihood of 0.011 (ΔAIC=9.05, AIC weight=0.008). Thus, the IDH was supported both for total disturbance (including perpetual disturbance) and for temporary disturbance alone, suggesting the hypothesis is robust to disturbance permanence. Our results for native species in anthropogenically disturbed communities lend support to the IDH, in contrast to more than 80% of other studies that did not exhibit the predicted unimodal relationship [4] , [5] . We attribute support for IDH found in this study but not many others to several aspects of study design. First, our study was conducted at a large regional extent. Reviews of IDH concluded many tests of IDH have been inadequately small scaled [4] , [5] , [8] ; few tests have approached the regional extents at which the IDH was intended to apply (for example, the 35,000-ha Budongo rainforest [3] ). Connell [3] , who advanced the IDH, was specific in stating this hypothesis applied to 'variation in diversity among local stands (that is, communities)', not among sites within small communities nor among large biomes. Diversity–disturbance relationships at either local (for example, within a single community) or interregional scales are generated by different processes and tend to exhibit different diversity patterns [16] . Our study was truly regional because we observed consistent results among widely separated communities sampled across a large geographic range. Second, we utilized a direct measure of disturbance: area altered by human land use. Data-rich studies of tropical forest trees [8] , [17] , [18] have used indirect proxies for disturbance such as % pioneer species or canopy height, which may have contributed to their opposing conclusions and which have been criticized for their poor interpretability [7] . Third, the communities under investigation varied on a full gradient of 0–100% disturbance extent. Many studies may have encompassed a narrow range of disturbance levels, thereby risking missing any 'intermediate' peak in richness [4] , [5] , [8] . Our results have important implications for prominent theories of species invasion, which predict a strong link between richness of native and exotic species. Communities richer in native species may be more resistant to invasion of exotics due to competition among species, thereby producing a negative relationship between native and exotic richness [19] , [20] , [21] . A contrasting idea suggests native and exotic species richness should be positively related because the key environmental factors driving richness are shared by native and exotic species [22] , [23] . We found little support for either of these conflicting predictions: native species ( x ) weakly explained exotic ( y ) richness ( y =0.030 x +1.440, r 2 =0.033, P =0.005). By contrast, human disturbance was a relatively good predictor of exotic richness ( r 2 =0.371, P <0.001), supporting the view that exotic species are not independent drivers of native biodiversity declines, but 'passengers' simply accompanying community change in disturbed environments [24] . Considerations of biodiversity conservation in regional land use planning decisions usually focus on preservation of species, which are at risk or have particular economic or cultural value. However, biodiversity is increasingly being more broadly considered in land use planning decisions [25] , species richness is considered in conservation prioritization [26] and ecological theory is being called upon to aid conservation-oriented land use decisions [27] . We show that the IDH can partially explain the variation in species richness found throughout a large region subjected to a diversity of anthropogenic impacts. Although simple, IDH is an enduring idea that may be applicable to land use planning [28] and along with invasion theories can contribute to understanding changes in native richness expected with human land use [29] . Our results are generally consistent with both the IDH and the more specific 'patch mosaic dynamics hypothesis', which suggests that landscapes with a mosaic of disturbed patches of various intensity, extent and frequency can host the greatest diversity [30] . However, our findings also suggest that management strategies designed to maximize biodiversity by imposing intermediate human disturbance regimes could result in communities with species composition statistically indistinguishable from those at high disturbance ( Fig. 3 ), exclusion of some species or community types found only at low disturbance, and proportionally fewer native species [29] ( Fig. 4b ). Thus, we strongly suggest any management application of this work takes into consideration the overall species composition across the study area, and not focus solely on species richness levels in individual plots. As disturbance was more strongly correlated with and better predicted richness of exotics than natives, management efforts aimed exclusively at maximizing species richness could have a greater impact on exotic species than natives. We found that although human disturbance significantly predicted native species richness ( r 2 =0.104, P <0.001), the interactive effects of disturbance and exotic species richness explained nearly twice as much variation in native richness as did disturbance alone ( r 2 =0.206, P <0.001). Efforts to conserve native species diversity should therefore consider not only management of human disturbance but also the interactions of land use and exotic species, such as the roles of human disturbance in creating opportunities for exotic species establishment or acting as conduits for exotic dispersal [29] , [31] . Catford et al . [29] suggest a range of management options informed by IDH and invasion patterns. However, the inconsistency in support and possible scale dependence of IDH warrant caution in its application. In the boreal biome, among the world's largest and most intact terrestrial ecoregions, the IDH may serve as a starting point for understanding how continued expansion of human activities may affect local plant communities. Study design Vascular plant richness was surveyed in the boreal ecoregion of the province of Alberta, Canada by the Alberta Biodiversity Monitoring Institute, using standardized protocols [32] . Vascular plant species occupancy was surveyed within 1 ha for 25 min at 242 sites, a subset of 959 sites of the Canadian National Forestry Inventory grid with grid centre spacing of 20 km ( Fig. 1 ). All surveys were conducted from 26 June to 18 August of 2003–2009. Human disturbance extent (% land area converted by humans) was assessed by manual interpretation of 1:30,000 aerial photos and SPOT satellite imagery within circles of 150 m radius (7.07 ha) at each site. Disturbance extent was assessed within a larger area than that at which richness was surveyed, because both direct local disturbances and those in the surrounding landscape may potentially affect local richness [33] . We distinguished native and exotic species according to ACIMS [34] . To determine the best-fit shape of the richness–disturbance relationship, we performed linear and polynomial regression analyses. Polynomial (quadratic and cubic) models required additional model parameters not included in simple linear regression, so we adopted those models only when they were both significant (reported as ' P <0.05') and when they fit significantly better by explaining significantly more variation than the simpler model of fewer parameters, as diagnosed with an ANOVA of candidate models (reported as ' P of increase in r 2 over linear model'). In all cases, that frequentist model selection protocol resulted in the same adopted model as with model selection by AIC (highest model likelihood, AIC weight >0.5). Disturbance types Human disturbance only described spatial extent of disturbance; it was not a measure of 'area removed' (as in some theoretical models) and we did not quantify intensity, frequency or time as disturbance, which varied greatly within and among disturbance types. Anthropogenic disturbances included agricultural pasture and croplands, forestry cut areas of variable ages, linear features (including pipelines, powerlines, roads, railways and cutlines primarily for oil/gas seismic exploration), industrial/commercial disturbances (including coal and mineral surface mines, oil and gas well pads, communication towers, gravel pits, heavy oil sands development and spoil piles), and both urban and rural settlements. Natural disturbances such as fire and insect damage were not correlated to anthropogenic disturbance. Species composition To determine if species composition of communities was consistent with proposed mechanisms for the IDH, we tested for differences in species composition among communities varying in human footprint. We classified sites as <33.3, 33.4–66.6 and >66.7 human footprint and used a multi-response permutation procedure using a Euclidean distance measure and rank-transformed distance matrix to make pairwise comparisons of species composition across sites grouped by human footprint class. We performed non-metric multidimensional scaling analysis, an ordination technique that graphically presents the overlap in composition across sites, then classified each site by disturbance level ( Fig. 3 ). Species origin and growth form We used a common non-taxonomic categorization of plant species—'growth form'—to explore the consistency of the IDH among species of different functional types [14] . Vascular plant species in boreal Alberta vary from small herbaceous forbs to tall woody canopy trees, and because these different growth forms have different functional roles, they could be expected to respond differently to disturbance [35] . Environmental covariates To determine the best-fit shape of the richness–disturbance relationship while accounting for potentially confounding variables, we constructed multiple regression models and selected model shapes as above. For human disturbance and each environmental covariate, we selected the best fitting linear or polynomial form. We used a subset of 146 sites for which data was available for 18 potentially confounding variables. We included in the models human disturbance plus the following: natural subregion type, latitude, longitude, elevation, topographic heterogeneity, growing degree days, mean annual temperature, mean annual precipitation, terrain wetness, site wetness, solar flux, canopy closure, oldest tree age, organic depth, soil type, surficial geology, slope position and landform classification ( Supplementary Table S4 ). Too few data were available to include natural disturbance (year of last fire and natural disturbance extent) in the models. Details of environmental variable observation and estimation are available at www.abmi.ca . Temporary anthropogenic disturbance To investigate the relationship of richness to temporary disturbance, we categorized forestry cut areas, cutlines, pipelines and powerlines as temporary, and all other disturbances as perpetual. We first excluded all sites with any perpetual disturbance at the 1-ha scale where vascular plants were sampled. We then subtracted any perpetually disturbed area in the 150-m radius circle plot and calculated the proportion of temporary disturbance in the remaining area. How to cite this article: Mayor, S.J. et al . Regional boreal biodiversity peaks at intermediate human disturbance. Nat. Commun. 3:1142 doi: 10.1038/ncomms2145 (2012).